Scalable-produced 3D elastic thermoelectric network for body heat harvesting 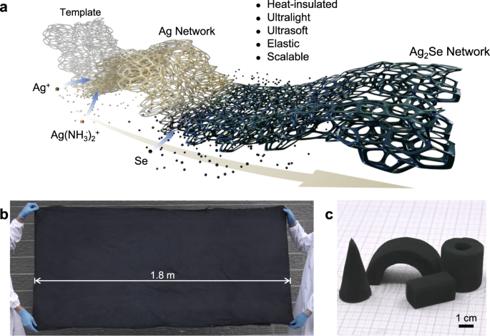Fig. 1: Fabrication process and photos of Ag2Se network. aSchematic of the two-step impregnation process, showing the in-situ synthesis of Ag2Se network by silvering and then selenizing.bA large Ag2Se network with a size of 1.8 × 0.9 m2.cAg2Se networks are processed to special shapes. Flexible thermoelectric generators can power wearable electronics by harvesting body heat. However, existing thermoelectric materials rarely realize high flexibility and output properties simultaneously. Here we present a facile, cost-effective, and scalable two-step impregnation method for fabricating a three-dimensional thermoelectric network with excellent elasticity and superior thermoelectric performance. The reticular construction endows this material with ultra-light weight (0.28 g cm −3 ), ultra-low thermal conductivity (0.04 W m −1 K −1 ), moderate softness (0.03 MPa), and high elongation (>100%). The obtained network-based flexible thermoelectric generator achieves a pretty high output power of 4 μW cm −2 , even comparable to state-of-the-art bulk-based flexible thermoelectric generators. With the rapid development of “Internet of Things” technology, the popularity of flexible electronics has risen enormously. As a result, the global flexible electronics market was valued at USD ~28 billion in 2020 and that is expected to reach USD ~ 56 billion by 2026 [1] . However, the convenience and endurance of the most common flexible electronics are hindered by their power sources which need to be able to operate continuously [2] . Various energy-harvesting technologies, such as triboelectric nanogenerators [3] , [4] , piezoelectric nanogenerators [5] , flexible solar cells [6] , [7] , and flexible thermoelectric generators (FTEG) [2] , [8] , were thus developed. Features that directly convert body heat into electricity make the FTEG highly appealing, as power is sustainably generated without the need for chemical energy, sunlight, or mechanical motion [9] , [10] , [11] . The common bulk thermoelectric materials, whether inorganic materials (e.g., bismuth antimony telluride alloys [12] and silver selenide [13] , etc.) or conducting polymers [e.g., PEDOT:PSS (poly (3,4-ethylenedioxythiophene):poly (styrene sulfonate)) [14] , [15] , [16] and PANI (polyaniline) [15] , [17] , [18] , [19] ], are intrinsically inflexible [20] . Some strategies were thus proposed to meet the flexibility of FTEG. One strategy is processing the thermoelectric material into thin film or sheet [21] , [22] , [23] , [24] , [25] , [26] , [27] , [28] , [29] . Although bendable [26] , [27] , [30] or even elastic [31] , the thermoelectric thin film or sheet usually harvests thermal energy in the in-plane direction rather than in the more desirable film-thickness direction. Three-dimension (3D) FTEG, by contrast, is more suitable for harvesting body heat during wear. Combining flexible matrix with rigid thermoelectric legs is a device-level strategy to obtain 3D FTEGs [32] , [33] , [34] , [35] , [36] , [37] . This kind of FTEG has the highest thermoelectric performance, but the heavy and incompatible rigid thermoelectric legs significantly reduce their wearing comfort and reliability [9] , [38] . To better match the elastic skin, improve comfortability, and recover the deformation induced in operation, developing a thermoelectric material with elasticity is necessary for an FTEG. Mixing insulating elastomers with conducting polymers or carbon nanotubes can result in 3D stretchable thermoelectric materials or thermoelectric elastomers [18] , [20] , [39] , [40] , [41] . However, these composites demonstrate inferior thermoelectric performance ( zT < 0.03) in comparison to the inorganic thermoelectric materials due to their intrinsically low Seebeck coefficient [20] . Consequently, achieving a material simultaneously possesses elasticity and high thermoelectric performance is still challenging. Here, we report a facile, cost-effective, and scalable two-step impregnation method for synthesizing a 3D Ag 2 Se network. Benefiting from the deformable and low-thermal-conductive network structure, the proposed thermoelectric network can not only exhibit sufficient elasticity (elongation > 100%), but also achieve a comparable output power to traditional bulk-based FTEGs with the flexible matrix. Unlike the conventional preparation process of thermoelectric material or device, our fabrication technique depends hardly on complex equipment, which makes the Ag 2 Se network can be large-scale produced at low cost and processed into special shapes to match the various heater surfaces. Furthermore, the soft texture (Young’s modulus ~0.03 MPa) and the ultralight weight (density ~0.28 g cm −3 ) of Ag 2 Se network also ensure its enormous potential in wearable applications. A thermoelectric network-filled jacket is fabricated to verify the actual effect of body heat harvesting. It can generate milliwatt-level power in daily wear, covering the consumption of most integrated circuits and sensors in wearables [42] , [43] . The high output performance, scalable technique, and significant advantages in wearability enable the promising applications of Ag 2 Se network. Three-dimensional elastic Ag 2 Se network Our two-step impregnation method for making the Ag 2 Se network (Fig. 1a ) is inspired by two classical chemical reactions, “Tollens’ reaction” [44] and “Transition metal selenization” [45] . In the first step, SnCl 2 -pretreated melamine template is immersed into Tollens’ reagent containing Ag + and Ag(NH 3 ) 2 + . The Ag + in the solution is reduced by the Sn 2+ on the template to form Ag nucleus [46] , and the coexisting Ag(NH 3 ) 2 + is subsequently reduced by the reductant comprising glucose monohydrate and potassium sodium tartrate tetrahydrate to form a silver network. In the second step, the obtained silver network is impregnated into the selenium solution [47] for selenizing to in-situ synthesize the Ag 2 Se network [48] . The porosity of the Ag 2 Se network measured with the Archimedes method can be controlled from 98% to 95% with a pristine porosity of 99% through the adjustment of reaction proportion and reaction times (Fig. S1 ). The detailed optimization is provided in Experimental Section. Because all the procedures are handled at ambient conditions, a nearly 2-square-meter sample is effortlessly produced (Figs. 1b and S3 ). Furthermore, unlike brittle thermoelectric bulks, the obtained three-dimensional network can be easily processed into special shapes (e.g., arch, cone, cuboid, and tube, etc.) to match well with the complex heater surfaces (Fig. 1c ). Fig. 1: Fabrication process and photos of Ag 2 Se network. a Schematic of the two-step impregnation process, showing the in-situ synthesis of Ag 2 Se network by silvering and then selenizing. b A large Ag 2 Se network with a size of 1.8 × 0.9 m 2 . c Ag 2 Se networks are processed to special shapes. Full size image With the help of the micro-scale structure deformation, the Ag 2 Se network demonstrates macro-scale stretching and compressing (Fig. 2a–c ), which is similar to the metal-mesh electrodes characterized in the previous works [49] . A tensile strain ( ε t ) of >100% and a compressive strain ( ε c ) of >80% were obtained (Fig. 2d ). The Young’s modulus of the Ag 2 Se network extracted from the compressive stress-strain curve is ~0.03 MPa, which is considered as an ideal and tissue-like modulus that enables the intimate fitting of devices with the uneven skin, reducing the effects of mechanical loads [50] , [51] , [52] , [53] . The room-temperature Seebeck coefficient and resistivity of the Ag 2 Se network under compressive and tensile strains were measured on a ZEM-3. The results indicate that there is little change in the Seebeck coefficient with the strain, and the change in power factor mainly results from the change in resistivity, which can be ascribed to the variation in the geometric size of the Ag 2 Se network. (Fig. S4 ). We also carried out cyclic mechanical and electromechanical tests to show the durability of the Ag 2 Se network (Fig. 2e–g ). Even though a hysteresis in the stress-strain curve is observed because of viscoelasticity, the sample can recover to its initial state after the successive cycles at different strains (Fig. 2e ). A slight mechanical degradation occurs in the initial cycle of the tensile-strain test (Fig. 2f ), but it does not deteriorate in the subsequent cycles. Correspondingly, the relative resistance of the Ag 2 Se network almost remained stable under cyclic tests with different strain rates (Fig. 2g ). The changes in resistance are similar to the typical trend of stretchable conductive materials [31] , [54] . The possible reasons for the decline in resistance over cycles are the alignment of fibrils and the viscoelasticity of the template [31] , [55] . The Ag 2 Se network, as an elastic material, also performs well in bending. It can survive 200 cycles bending with a 5 mm radius without significant deterioration (Fig. S5 ). Additional characterizations of the Ag 2 Se network including morphology, energy dispersive spectrum, element mapping, XRD pattern, and optical bandgap are provided in Fig. S6 – S10 and Table S1 . The obtained Ag 2 Se network is a single phase without any impurity, and the bandgap is about 0.23 eV. Fig. 2: Mechanical, and thermoelectric properties of Ag 2 Se network. a – c Photos (inset) and cross-section micrographs of the Ag 2 Se network in different states, showing the deformation of network structure under stress. d Tensile stress ( σ t )–strain ( ε t ) curve and compressive stress ( σ c )–strain ( ε c ) curve with corresponding resistance change ( R / R 0 ). e Cyclic σ c – ε c curves with strain varying from 50% to 80% (bottom left), and σ t – ε t curves with strain from 40% to 100% (top right). f Cyclic strain-stress curves at a maximum ε c of 80% (bottom left) and a maximum ε t of 100% (top right). g R / R 0 upon cyclic compressing (top) and stretching (bottom) under different strain rates. h Thermoelectric performance of Ag 2 Se network including electrical resistivity ( ρ ), Seebeck coefficient ( S ), power factor ( PF ), and zT value. i Comparison of the present zT value with reported 3D flexible thermoelectric materials. The inset shows the larger version of the zT values of CNT-based materials. Error bars represent the standard deviation. Source data are provided as a Source Data file. Full size image Together with good mechanical properties, the Ag 2 Se network also possesses superior thermoelectric performance (Fig. 2h ). It displays a similar Seebeck coefficient (~−130 μV K −1 ) and much lower thermal conductivity (~0.04 W m −1 K −1 , Fig. S11 ) compared with that of Ag 2 Se bulk materials at room temperature [56] , [57] . A high room-temperature zT ~ 0.11 is achieved, which is one or two orders of magnitude higher than the previously reported three-dimensional flexible thermoelectric materials based on polymer composites [18] , [40] , [41] , [58] , [59] , [60] , [61] , [62] , [63] , [64] , [65] (Fig. 2i ), indicating that structuring inorganic material is also another viable pathway to develop three-dimensional flexible thermoelectric materials. Ag 2 Se network-based device The ultralow thermal conductivity of the Ag 2 Se network is highly desirable for the FTEG. First, it endows the FTEG with a superior ability to establish temperature difference, unlike the bulk-based FTEG, which has to enlarge the temperature difference by increasing the leg height, decreasing the fill factor (the percentage of total FTEG area occupied by the thermoelectric legs) or imposing a heat sink. This advantage is native to the network-based FTEG without additional weight, volume, or power. By finite element simulation, we compared the temperature distribution between the network-based FTEG, the full-filled bulk-based FTEG and the 10% filled FTEG at the same thickness of 3 mm (Fig. 3a–c ). The completely filled and 10% filled bulk-based FTEGs are made up of Bi 2 Te 3 -based thermoelectric legs and PDMS (Polydimethylsiloxane) matrix, which are common in the previous works [66] , [67] . The network-based FTEG shows a large temperature difference of ~6.5 K, one order higher than the full-filled bulk-based FTEG and three times higher than the 10% filled FTEG. Second, the Ag 2 Se network-based FTEG can maintain normal body surface temperature during operation, which is essential but often unconsidered. To maximize the output power, it is better to use FTEGs in a cold environment. Suffering from the high thermal conduction or the heat sink cooling, the temperature drop in body surface caused by the low hot-side temperature is a significant complication for bulk-based FTEG, which can be avoided in the network-based FTEG as its interior low thermal conduction can prevent heat loss. According to the simulated temperature field (Fig. 3a–c ), the network-based FTEG’s hot side temperature (~304 K) is closer to skin temperature (306 K) than the bulk-based FTEGs. We also compared the output performance by simulation at different ambient temperatures from 273 K to 305 K (Fig. 3d, e ). A great increase in the open-circuit voltage of the network-based FTEG appears in comparison to the bulk-based FTEGs due to the larger temperature difference (Fig. 3d ). Consequently, the power density (output power per unit area) of the network-based FTEG is similar to that of the 10% filled FTEG (Fig. 3e ). The infrared image of the network-based FTEG wore on the arm experimentally demonstrates the obvious low temperature on the Ag 2 Se network’s surface (Fig. 3f ). Although the tested voltage and power density of a network-based FTEG attached on the arm are slightly lower than the simulated results (Fig. 3g, h ), which is because of the contact resistance, the power density of network-based FTEG is several order higher than that of PEDOT- or CNT-based FTEGs and is even on par with high-performance bulk-based FTEGs [25] , [29] , [32] , [37] , [66] , [68] , [69] , [70] , [71] , [72] , [73] (Fig. 3i ). Additionally, the device demonstrates excellent reliability and can operate continuously for 50 h without degradation in output performance (Fig. S12 ). Fig. 3: Output performance of Ag 2 Se network-based FTEG. The simulated internal temperature distribution of the full filled ( a ), 10% filled ( b ) bulk FTEGs and the network-based FTEG ( c ) at an ambient temperature of 290 K. Further simulation details are provided in the supplementary materials. d , e , The simulated single leg voltage and power density in an ambient temperature range from 273 K to 305 K. f The infrared image and optical photograph (inset) of a network-based FTEG dressed on a human wrist. The top electrode was removed to avoid the effect caused by its low emissivity. g , h The measured voltage and power density at an ambient temperature of 290 K and 297 K. Inset shows a device under test. i Summary of the FTEG’s power generation at different ambient temperatures. All the measurements were performed on human skin without heat sinks. Red line and red circles respectively represent the simulated and measured values of the Ag 2 Se network-based FTEG. Source data are provided as a Source Data file. Full size image The excellent output performance of network-based FTEG is complemented by portability and scalability, which encourages us to take one step further toward FTEG’s practical use. We replaced a portion of the filler (20 × 20 cm 2 ) in a commercial jacket with the network-based FTEG with 40 legs in series to verify the actual effect (Fig. 4a–c and Fig. S15 ). Promisingly, most of the device’s performance can be preserved even under such a non-ideal condition including the presence of hand-arranged module gaps, and the untight touching between the module’s hot side and skin surface (Fig. 4, d, e ). When the wearer was sitting stationary in an indoor environment at 290 K, the maximum power of the thermoelectric jacket was ~0.6 mW. The output power increased to ~1 mW when the wearer was walking at a speed of 1 m s −1 . In addition, although the thermal bypass in the current configuration of the FTEG module based on one-type TE leg has a negligible effect on the temperature difference (Fig. S16 ), the increased internal resistance is inevitable. 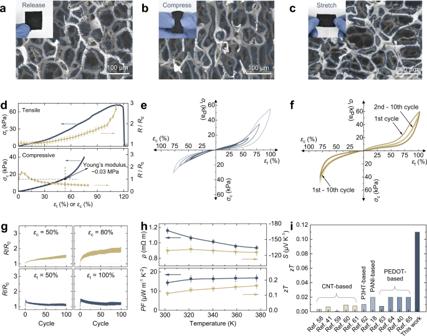Fig. 2: Mechanical, and thermoelectric properties of Ag2Se network. a–cPhotos (inset) and cross-section micrographs of the Ag2Se network in different states, showing the deformation of network structure under stress.dTensile stress (σt)–strain (εt) curve and compressive stress (σc)–strain (εc) curve with corresponding resistance change (R/R0).eCyclicσc–εccurves with strain varying from 50% to 80% (bottom left), andσt–εtcurves with strain from 40% to 100% (top right).fCyclic strain-stress curves at a maximumεcof 80% (bottom left) and a maximumεtof 100% (top right).gR/R0upon cyclic compressing (top) and stretching (bottom) under different strain rates.hThermoelectric performance of Ag2Se network including electrical resistivity (ρ), Seebeck coefficient (S), power factor (PF), andzTvalue.iComparison of the presentzTvalue with reported 3D flexible thermoelectric materials. The inset shows the larger version of thezTvalues of CNT-based materials. Error bars represent the standard deviation. Source data are provided as aSource Datafile. To further enhance the output power, a thick electrode would be utilized in this module, resulting in the larger thermal bypass. 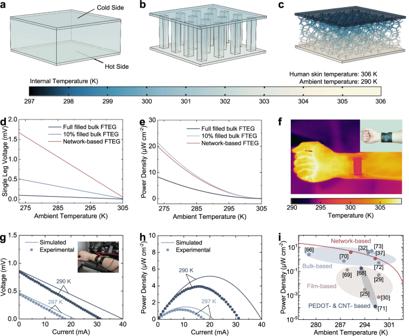Fig. 3: Output performance of Ag2Se network-based FTEG. The simulated internal temperature distribution of the full filled (a), 10% filled (b) bulk FTEGs and the network-based FTEG (c) at an ambient temperature of 290 K. Further simulation details are provided in the supplementary materials.d,e, The simulated single leg voltage and power density in an ambient temperature range from 273 K to 305 K.fThe infrared image and optical photograph (inset) of a network-based FTEG dressed on a human wrist. The top electrode was removed to avoid the effect caused by its low emissivity.g,hThe measured voltage and power density at an ambient temperature of 290 K and 297 K. Inset shows a device under test.iSummary of the FTEG’s power generation at different ambient temperatures. All the measurements were performed on human skin without heat sinks. Red line and red circles respectively represent the simulated and measured values of the Ag2Se network-based FTEG. Source data are provided as aSource Datafile. 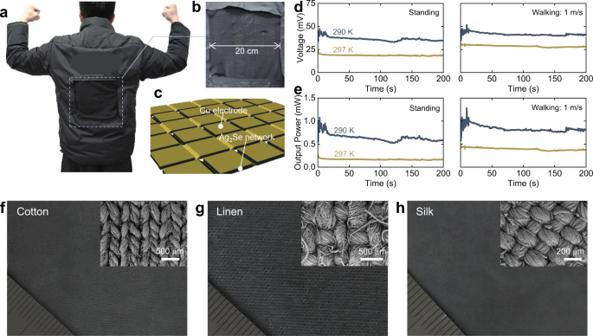Fig. 4: Thermoelectric jacket and fabrics. aA thermoelectric jacket filled with the Ag2Se network-based FTEG.bDetailed photograph of the thermoelectric-device area.cSchematic of the thermoelectric modules in series.d,eThe thermoelectric jacket’s open-circuit voltage and output power under different thermal conditions.f–hThe optical photos and morphologies (inset) of various thermoelectric fabrics. Further micrographs and thermoelectric performances are shown in Figs.S13andS14. Ruler scale unit: mm. Source data are provided as aSource Datafile. We assembled the device with two p-type Bi 2 Te 3 -based legs and two n-type Ag 2 Se-based networks (Device size: 4.1 × 2.6 cm 2 ) to estimate the possible performance of the device, and the tested results are shown in Fig. S17 . As expected, the TEG with an n-p design exhibits higher performance. A voltage of ~15 mV and a power density of ~1.7 μW cm −2 can be reached, even if its geometric is not particularly optimized, exceeding the performance of the presented single-leg device (with a voltage of ~0.44 mV and a power density of ~1.2 μW cm −2 ) at the same ambient temperature of 297 K. However, the weight and portability of the TEG with rigid p-type Bi 2 Te 3 would have deteriorated in comparison with the network-based device. Consequently, developing matched flexible p-type materials is really necessary. Fig. 4: Thermoelectric jacket and fabrics. a A thermoelectric jacket filled with the Ag 2 Se network-based FTEG. b Detailed photograph of the thermoelectric-device area. c Schematic of the thermoelectric modules in series. d, e The thermoelectric jacket’s open-circuit voltage and output power under different thermal conditions. f – h The optical photos and morphologies (inset) of various thermoelectric fabrics. Further micrographs and thermoelectric performances are shown in Figs. S13 and S14 . Ruler scale unit: mm. Source data are provided as a Source Data file. Full size image The two-step impregnation method, shown here for the Ag 2 Se network, can also be applied to fabric substrates, including cotton, linen, and silk (Fig. 4f–h and Figs. S11 , S18 , S19 ). The technique thus allows ordinary cloth or clothing to be easily processed into personalized thermoelectric devices for the power supply or thermoregulation. The diverse possibilities enable the two-step impregnation technique, a universal strategy for making wearable thermoelectric products. Additionally, some compatible techniques or materials are deserved to be investigated. For instance, substituting liquid metal electrodes for copper electrodes to meet the Ag 2 Se network’s elasticity, and developing p-type thermoelectric materials using similar techniques to pair with n-type Ag 2 Se. Preparation of the three-dimensional Ag 2 Se network and the network-based FTEG Template preprocessing A high-density melamine foam (Basotect; BASF) was first rinsed in NaOH solution (80 g/L) for 30 min, and then cleaned with deionized water. Tin (II) chloride dihydrate (SnCl 2 ·2H 2 O, 98%; Innochem) was dissolved in deionized water (40 g/L) to make Sn 2+ solution, followed by the addition of hydrochloric acid (AR; Xilong Scientific) until the solution is clear. The template was then immersed into Sn 2+ solution for 2 h and transferred into deionized water for rinsing. Finally, the treated template dried naturally. Silvering Glucose monohydrate (C 6 H 12 O 6 ·H 2 O, AR; Hushi), potassium sodium tartrate tetrahydrate (C 4 H 4 O 6 KNa·4H 2 O, AR, 99%; Aladdin), and PEG1000 (CP, Hushi) were dissolved in a diluted ethanol solution to make a reductant. The concentrations of C 6 H 12 O 6 ·H 2 O, C 4 H 4 O 6 KNa·4H 2 O, PEG1000, and ethanol were 40 g/L, 14 g/L, 0.1 g/L, and 100 g/L, respectively. The Tollens’ reagent was prepared by dissolving silver nitrate (AgNO 3 , 98%; TBHX) and sodium hydroxide (NaOH, AR; Xilong Scientific) in an ammonium hydroxide solution (AR; Macklin). The aforementioned template was impregnated into the mixture of reductant and Tollens’ reagent, and squeezed gently to extrude the residual bubbles. After soaking for 5 h, the obtained silver network was washed and dried. It should be pointed out that the reaction rate and the number of reaction times will affect the silver loading and further influence the Ag 2 Se loading. Therefore, we adjusted the silver load by changing ammonia concentration and reaction times with a fixed AgNO 3 concentration of 50 g/L and NaOH concentration of 25 g/L (Fig. S1 ). Selenization To prepare the selenium solution, sodium sulfide nonahydrate (Na 2 S·9H 2 O, 98%; Aladdin) and selenium powder (Se, 99.9%; Innochem) were dissolved into deionized water with concentrations of 60 g/L and 20 g/L, respectively. The above-mentioned silver network was then impregnated into the selenium solution for 10 h to synthesize the Ag 2 Se network. Considering the reaction efficiency, the subsequent samples were prepared based on an ammonia concentration of ~4.5 mol/L and two repetitions. The color changes in reaction process are shown in Fig. S2 . The large-scale preparation was carried out in a polypropylene tank with a size of 2000 × 1000 × 100 mm 3 . Fabrication of the network-based FTEG The 10 μm-thick copper foils were used as electrodes, connected with the Ag 2 Se networks by silver paste (05002; SPI). A FTEG module including 40 thermoelectric legs of the Ag 2 Se networks was prepared in series, which was utilized to assemble a thermoelectric network-filled jacket by partially replacing the jacket’s filler. Characterization of the material and device Material characterization The porosity of the Ag 2 Se network was measured based on the Archimedes method by a density balance (BSA224S-CW; Sartorius). Morphology and energy dispersive spectrum of the Ag 2 Se network were observed by field emission scanning electron microscopy (Gemini Crossbeam 350; ZEISS). The crystal structure was determined by X-ray diffraction (SmartLab; Rigaku) using Cu Kα radiation in the 2 θ range of 10–70° at 40 kV and 200 mA. The mechanical properties were tested by a stress–strain apparatus (HTS-LLY920C; Zhongye). The Seebeck coefficient ( S ) and electrical resistivity ( ρ ) of Ag 2 Se networks with or without strain were measured simultaneously on a commercial system (ZEM-3; Advance Riko). The room-temperature thermal conductivity ( κ ) was determined by the hot wire method on a thermal conductivity meter (TC3000E; XIATECH). The given results are the mean of three measurements taken from the same sample. Optical bandgap was obtained on a Fourier transform IR reflectance spectrometer (Nicolet iS50; Thermo Fisher Scientific) equipped with an integrating sphere coated with gold (Pike). Simulation The output performance for the bulk-based and network-based FTEGs was simulated using the thermoelectric module in COMSOL. All simulations were performed under natural convection conditions (Fig. S13 ). We also calculated the open-circuit voltage ( U ) and power density ( p ) of the network-based FTEG with different thicknesses. According to the simulated results (Fig. S14 ), a module thickness of 3 mm was adopted in the experiments. The material parameters used in the simulation were summarized in Table S2 . Network-based FTEG characterization The output properties were measured in homemade equipment connected with two electricity meters (2400 and 2182; Keithley). The IR image was captured using a thermal IR imager (T620; FLIR). The ambient temperature and wind speed were recorded by a portable weather station (PWS; Qingyi). Ethics and inclusion statement The authors declare that their study was approved by Harbin Institute of Technology (Protocol number: HIT-2022012), and they have obtained informed consent for publication from all participants. Reporting summary Further information on research design is available in the Nature Portfolio Reporting Summary linked to this article.